Role of motor cortex NMDA receptors in learning-dependent synaptic plasticity of behaving mice The primary motor cortex has an important role in the precise execution of learned motor responses. During motor learning, synaptic efficacy between sensory and primary motor cortical neurons is enhanced, possibly involving long-term potentiation and N-methyl-D-aspartate (NMDA)-specific glutamate receptor function. To investigate whether NMDA receptor in the primary motor cortex can act as a coincidence detector for activity-dependent changes in synaptic strength and associative learning, here we generate mice with deletion of the Grin1 gene, encoding the essential NMDA receptor subunit 1 (GluN1), specifically in the primary motor cortex. The loss of NMDA receptor function impairs primary motor cortex long-term potentiation in vivo . Importantly, it impairs the synaptic efficacy between the primary somatosensory and primary motor cortices and significantly reduces classically conditioned eyeblink responses. Furthermore, compared with wild-type littermates, mice lacking NMDA receptors in the primary motor cortex show slower learning in Skinner-box tasks. Thus, primary motor cortex NMDA receptors are necessary for activity-dependent synaptic strengthening and associative learning. The primary motor cortex (M1) is pivotal for sensorimotor integration and precise control of voluntary movements [1] . Sensory signals in the cortex are represented as activity maps, with active neurons organized as functional clusters or modules [2] , [3] , which are continuously re-shaped by experience and learning [4] , [5] , [6] , [7] . However, there are also dynamic interactions between widely distributed functional modules in different cortical and subcortical regions. These interactions, by way of ‘putative’ overlapping functional neuronal assemblies [8] , are thought to form the necessary neural substrates for multimodal processing, and learning and memory consolidation [9] . At a connectivity level, cortical excitatory neurons, with their elaborate basal and apical dendrites, receive synaptic input from distantly located excitatory neurons, and local excitatory as well as inhibitory neurons [10] . Reciprocal corticocortical connections [11] and functional interactions between M1 and the primary somatosensory cortex (S1) [7] , [12] , possibly involving mechanisms of synaptic integration in different dendritic compartments [13] , [14] , with recruitment of N-methyl-D-aspartate (NMDA) receptor (NMDAR) channels [13] , are thus hypothesized to have an important role, for example, in organizing an animal’s motor activity plan to changes in the sensory experiences. In classical associative learning, neurons corresponding to variant sensory cues are linked together to form ‘memory’ representations. It has been hypothesized that cue–response associations occur in the M1 cortex, which enables an animal to make a correct sensory-guided behavioural response. Eyeblink conditioning (EBC) is a form of classical conditioning that is well suited to dissect the cellular and molecular mechanisms of learning and memory consolidation. In EBC, the conditioned stimulus (CS), such as a tone, is paired with the unconditioned stimulus (US), such as a mild shock, to the eyelid. In untrained animals, the US alone elicits an eyeblink as the unconditioned response (UR). However, after repetitive CS–US pairings, the CS alone is sufficient to elicit an eyeblink, or the conditioned response (CR). In the delayed EBC, the CS is presented before the US and the two stimuli end together. In the trace EBC, however, there is a stimulus-free period (trace interval) between the CS and the US. While both of these conditioning paradigms require the cerebellum [15] , the trace EBC also requires the participation of the hippocampus [16] , [17] and the cortex [18] , [19] . During motor learning, sensory signals are transmitted to the M1 cortex, inducing morphological and functional plasticity on multiple timescales [20] , [21] . Dynamic changes in neuronal activity [7] , [22] and activation of immediate-early genes [23] in the M1 cortex call into action cellular and molecular processes to strengthen pre-existing sensorimotor synaptic connections and to form new synapses [24] , [25] . The M1 cortex has the capacity for long-term potentiation (LTP) [26] , a candidate cellular model for learning and memory consolidation, and, importantly, LTP can be induced in this region by learning [27] . Recognizing the crucial role of NMDAR function in learning-induced cortical LTP [28] , map plasticity [29] and trace conditioning [30] , [31] , [32] , we hypothesized that the motor cortex NMDAR might act as a coincident detector for activity-dependent plasticity and associative learning. To test this hypothesis, we generated mice lacking GluN1 and hence NMDAR specifically in the M1 cortex ( Grin1- vΔ MCx ). Here we show for the first time that the NMDAR function in the M1 cortex is important for learning-dependent synaptic plasticity and acquisition of associative memory for both classical and instrumental conditioning paradigms. Cre-mediated Grin1 gene deletion To generate M1 cortex-specific Grin1 gene knockout mice, we developed a combinatorial genetic approach using viruses for conditional Cre recombinase ( Cre ) gene expression ( Fig. 1a ) in genetically engineered mice ( Grin1 tm1Rsp or Grin1 2lox ) [33] , in which exons of the Grin1 gene were flanked with loxP sites ( Fig. 1b ). We developed two recombinant adeno-associated viruses (rAAVs), which are equipped with the doxycycline (Dox)-controlled genetic switches [34] , [35] . The first virus ( rAAV-hSYN-rtTA ) allows expression of reverse tetracycline transactivator ( rtTA ) gene under control of the human synapsin promoter ( hSYN , Pro in the Fig. 1a ). The second virus ( rAAV-P tet bi-Cre/tdTOM ) is equipped with a bidirectional tet promoter ( P tet bi ) to simultaneously express two different genes encoding for the Cre recombinase protein and a red fluorescent protein variant, the tdTomato (tdTOM), for visualizing virus-targeted neurons ( Fig. 1a ). The Cre and the tdTOM genes are expressed when rtTA binds to P tet bi in the presence of Dox. To increase the spread of virus in the M1 cortex by hyperosmolarity, D-mannitol/virus mixture was injected in the brain [36] and D-mannitol was also delivered into mice systemically by intraperitoneal injection [37] ( Fig. 1c , Supplementary Fig. S1 ). Viruses were injected in the M1 cortex of age-matched wild-type littermates and Grin1 2lox mice [33] ( Fig. 1b ). Three weeks after virus injection, Dox-treated mice showed robust tdTOM and Cre expression in the M1 cortex ( Fig. 1c , Supplementary Fig. S2 ). Virus (v)-delivered Cre expression in neurons enabled, by Cre-loxP-mediated gene recombination, the generation of highly specific Grin1 gene knockout mice, Grin1 -vΔ MCx , in which the Grin1 gene is selectively deleted (Δ) in the M1 cortex (MCx) ( Fig. 1b,d ). The virus-injected, age-matched wild-type littermates served as controls ( Contr -v MCx ). 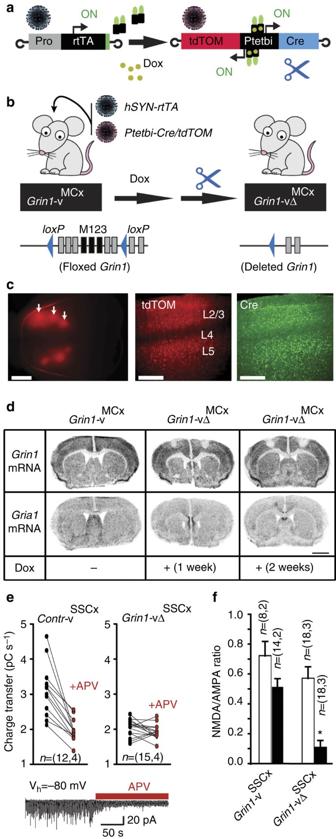Figure 1: Motor cortex-specificGrin1gene knockout. (a) Virus-mediated gene transfer for doxycycline (Dox) induced rtTA-dependent expression of tdTomato (tdTOM) and the Cre recombinase. (b) Cre expression in the brain ofGrin1tm1Rspmice (Grin12lox) activated the excision ofloxP-flanked exons in theGrin1gene, thereby generating mice with neuron-specificGrin1gene deletion selectively in the M1 cortex (Grin1-vΔMCx).LoxPsites, blue triangles; exons, grey rectangles; exons encoding membrane-inserted segments M1–M3, black rectangles. (c) Expression of tdTOM detected on both hemispheres with a three-point virus injection in the M1 cortex (scale bar; 3 mm, left). Cellular resolution tdTOM expression (scale bar; 250 μm, middle) and Cre (right) expression was specifically detected in cortical L2/3 and L5 (middle and right). (d)In situmRNA hybridization analyses revealed the absence ofGrin1mRNA expression in the M1 cortex ofGrin1-vΔMCxmice (with Dox for 1 week and 2 weeks), but not inGrin1-vMCxmice (without Dox). Expression ofGria1mRNA in the M1 cortex was detectable in bothGrin1-vMCxandGrin1-vΔMCxmice (Scale bar, 1 mm). (e) NMDAR-mEPSCs recorded atVh=−80 mV (sample trace at the bottom). NMDAR activity was detected by changes in charge transfer after 15 min of APV perfusion, measured over a time window of 125 s. 50 μM APV decreases charge transfer in cells ofContr-vSSCxmice, but notGrin1-vΔSSCxmice. A multiple comparison one-way ANOVA test was performed on four groups:Grin1-vΔSSCx;Grin1-vΔSSCx+APV;Contr-vSSCx; andContr-vSSCx, +APV mice (F3,49=24.11,P<0.001). (f) NMDA/AMPA ratios were averaged from sets of layer 2/3 pyramidal neurons recorded in either the left hemisphere (without virus injection, white bars) or right hemisphere (with virus injection, black bars). Ratios were similar between hemispheres from PBS-injected mice (seeSupplementary Fig. S5) and fromContrSSCxmice. However, inGrin1-vΔSSCxmice, there was a substantial decrease in the NMDA/AMPA ratio only in the virus-infected hemisphere (PBS or viruses were injected only on the right hemisphere) (Data from PBS injected animals is illustrated inSupplementary Fig. S5; F5,68=33.85, *P<0.05, multiple comparison one-way ANOVA). Error is presented as mean±s.e.m.n=(cells, mice). Figure 1: Motor cortex-specific Grin1 gene knockout. ( a ) Virus-mediated gene transfer for doxycycline (Dox) induced rtTA-dependent expression of tdTomato (tdTOM) and the Cre recombinase. ( b ) Cre expression in the brain of Grin1 tm1Rsp mice ( Grin1 2lox ) activated the excision of loxP -flanked exons in the Grin1 gene, thereby generating mice with neuron-specific Grin1 gene deletion selectively in the M1 cortex ( Grin1 -vΔ MCx ). LoxP sites, blue triangles; exons, grey rectangles; exons encoding membrane-inserted segments M1–M3, black rectangles. ( c ) Expression of tdTOM detected on both hemispheres with a three-point virus injection in the M1 cortex (scale bar; 3 mm, left). Cellular resolution tdTOM expression (scale bar; 250 μm, middle) and Cre (right) expression was specifically detected in cortical L2/3 and L5 (middle and right). ( d ) In situ mRNA hybridization analyses revealed the absence of Grin1 mRNA expression in the M1 cortex of Grin1 -vΔ MCx mice (with Dox for 1 week and 2 weeks), but not in Grin1 -v MCx mice (without Dox). Expression of Gria1 mRNA in the M1 cortex was detectable in both Grin1 -v MCx and Grin1 -vΔ MCx mice (Scale bar, 1 mm). ( e ) NMDAR-mEPSCs recorded at V h =−80 mV (sample trace at the bottom). NMDAR activity was detected by changes in charge transfer after 15 min of APV perfusion, measured over a time window of 125 s. 50 μM APV decreases charge transfer in cells of Contr -v SSCx mice, but not Grin1 -vΔ SSCx mice. A multiple comparison one-way ANOVA test was performed on four groups: Grin1 -vΔ SSCx ; Grin1 -vΔ SSCx +APV; Contr -v SSCx ; and Contr -v SSCx , +APV mice (F 3,49 =24.11, P <0.001). ( f ) NMDA/AMPA ratios were averaged from sets of layer 2/3 pyramidal neurons recorded in either the left hemisphere (without virus injection, white bars) or right hemisphere (with virus injection, black bars). Ratios were similar between hemispheres from PBS-injected mice (see Supplementary Fig. S5 ) and from Contr SSCx mice. However, in Grin1 -vΔ SSCx mice, there was a substantial decrease in the NMDA/AMPA ratio only in the virus-infected hemisphere (PBS or viruses were injected only on the right hemisphere) (Data from PBS injected animals is illustrated in Supplementary Fig. S5 ; F 5,68 =33.85, * P <0.05, multiple comparison one-way ANOVA). Error is presented as mean±s.e.m. n =(cells, mice). Full size image By in situ RNA hybridization (see Supplementary Methods ), we determined that the Grin1 mRNA was absent specifically in the M1 cortex of Grin1 -vΔ MCx mice (Dox-induced Grin1 gene deletion) ( Fig. 1d ). Virus-injected control mice, Grin1 -v MCx , (without Grin1 gene deletion) showed normal Grin1 mRNA expression ( Fig. 1d ). As expected, the expression of the Gria1 gene encoding the AMPA (α-amino-3-hydroxy-5-methyl-4-isoxazolepropionic acid) receptor (AMPAR) subunit 1 (GluA1) was unaffected in both groups of mice ( Fig. 1d ), and Nissl-staining revealed no observable loss of neurons due to virus injections ( Supplementary Fig. S3 ). NMDA receptor activity in acute brain slices As a proof-of-principle, we had arbitrarily targeted the somatosensory cortex (SSCx) for Grin1 gene deletion. We recorded NMDAR miniature excitatory postsynaptic currents (NMDAR-mEPSCs, see Methods) in acute brain slices prepared from Dox-treated control ( Cont -v SSCx , 12 cells, 4 mice) and Dox-induced Grin1 gene-deleted brain slices ( Grin1 -vΔ SSCx , 15 cells, 4 mice) ( Fig. 1e , Supplementary Fig. S4 ). We found that slices derived from Cont- v SSCx mice show large NMDAR-mEPSCs, which were blocked by the NMDAR-antagonist APV. However, charge transfer and NMDAR-mEPSCs were quite similar with and without APV in slices derived from the Grin1 -vΔ SSCx mice ( Fig. 1e , Supplementary Fig. S4 ). These results clearly demonstrate that NMDAR function is impaired in the Grin1 -vΔ SSCx mice ( Fig. 1e , Supplementary Fig. S4 ). As expected, Grin1 -vΔ SSCx mice also showed strong reduction in the NMDA/AMPA current ratios ( Fig. 1f , Supplementary Fig. S5 ). In vivo LTP measurements Initial in vivo experiments were aimed to determine the electrophysiological properties of S1–M1 synapses in behaving Grin1-vΔ MCx mice as compared with Cont -v MCx mice. Stimulating and recording electrodes were implanted in the corresponding facial areas of the primary somatosensory (S1) and motor cortices [18] ( Fig. 2a ). Both Cont- v MCx and Grin1 -vΔ MCx mice ( n =10 per group) presented similar (F (1,19,18) =2.310; P =0.145) increases in the slope of field excitatory postsynaptic potentials (fEPSPs) evoked at the M1 cortex following the presentation of single pulses of increasing intensity to the ipsilateral S1 region ( Fig. 2b ). These relationships were best fitted by sigmoid curves ( r ≥0.92; P <0.001), suggesting normal functioning of this synapse in both groups of mouse. In addition, no significant facilitation (or depression) of fEPSPs evoked during the paired-pulse test (F (5,54,48) =1.577; P =0.185) or significant (F (1,9,58) =0.000494; P =0.982) differences between the groups ( n =5 per group) were observed ( Fig. 2c ). These results indicate that the S1–M1 synapse does not present the paired-pulse facilitation typical of hippocampal synapses in behaving mice [38] and that no pre-synaptic changes [39] were evoked by deletion of the Grin1 gene. 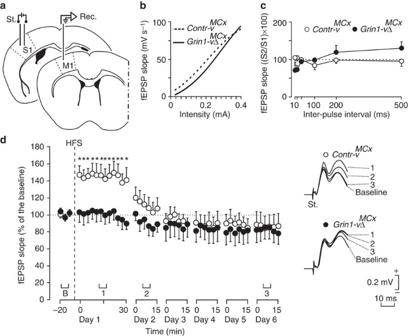Figure 2: Paired-pulse facilitation and long-term potentiation induction. (a) Schematic depicting electrode implantedin vivofor stimulating neurons in the S1 and recording in M1. (b) Input/output curves for the S1-primary motor cortex synapse. A single pulse was presented to S1 at increasing intensities (in mA), while recording the evoked fEPSP at the motor cortex forContr-vMCx(white circle and dashed line) andGrin1-vΔMCx(black circle and continuous line) mice. The best sigmoid adjustment to the collected data is represented (r>0.92;P≤0.001; non-linear regression analysis). There were no significant differences between groups (n=10 per group;P=0.145; F(1,19,18)=2.310; two-way ANOVA). (c) Responses to paired-pulse stimulation. The data shown are mean±s.e.m. slopes of the second fEPSP expressed as a percentage of the first for six (10, 20, 40, 100, 200 and 500) interstimulus intervals. The two groups (n=5 per group) of mice presented a similar (P=0.185; F(5,54,48)=1.577; two-way ANOVA) paired-pulse facilitation at intervals of 20–100 ms. (d) At the top are illustrated examples of fEPSPs collected from selectedContr-vMCx(white circles) andGrin1-ΔMCx(black circles) mice (n=10 per group) before (B, baseline) and after HFS of Schaffer collaterals. The bottom graphs illustrate the time course of LTP evoked in the motor cortex (fEPSP mean±s.e.m.) following HFS forContr-vMCxand Grin1-vΔMCxmice. The HFS was presented after 15 min of baseline recordings, at the time indicated by the dashed line. The fEPSP is given as a percentage of the baseline (100%) slope.Grin1-vΔMCxmice have no LTP. In addition, values collected from theContr-vMCxgroup were significantly (*P<0.01; F(6,54,63)=11.915; two-way ANOVA) larger than those collected fromGrin1-vΔMCxmice. Figure 2: Paired-pulse facilitation and long-term potentiation induction. ( a ) Schematic depicting electrode implanted in vivo for stimulating neurons in the S1 and recording in M1. ( b ) Input/output curves for the S1-primary motor cortex synapse. A single pulse was presented to S1 at increasing intensities (in mA), while recording the evoked fEPSP at the motor cortex for Contr -v MCx (white circle and dashed line) and Grin1 -vΔ MCx (black circle and continuous line) mice. The best sigmoid adjustment to the collected data is represented ( r >0.92; P ≤0.001; non-linear regression analysis). There were no significant differences between groups ( n =10 per group; P =0.145; F (1,19,18) =2.310; two-way ANOVA). ( c ) Responses to paired-pulse stimulation. The data shown are mean±s.e.m. slopes of the second fEPSP expressed as a percentage of the first for six (10, 20, 40, 100, 200 and 500) interstimulus intervals. The two groups ( n =5 per group) of mice presented a similar ( P =0.185; F (5,54,48) =1.577; two-way ANOVA) paired-pulse facilitation at intervals of 20–100 ms. ( d ) At the top are illustrated examples of fEPSPs collected from selected Contr -v MCx (white circles) and Grin1 -Δ MCx (black circles) mice ( n =10 per group) before (B, baseline) and after HFS of Schaffer collaterals. The bottom graphs illustrate the time course of LTP evoked in the motor cortex (fEPSP mean±s.e.m.) following HFS for Contr -v MCx and Grin1-vΔ MCx mice. The HFS was presented after 15 min of baseline recordings, at the time indicated by the dashed line. The fEPSP is given as a percentage of the baseline (100%) slope. Grin1 -vΔ MCx mice have no LTP. In addition, values collected from the Contr -v MCx group were significantly (* P <0.01; F (6,54,63) =11.915; two-way ANOVA) larger than those collected from Grin1 -vΔ MCx mice. Full size image Interestingly, the LTP study revealed significant differences between Grin1 -vΔ MCx and their littermate controls ( n =10 per group). Thus, high-frequency stimulation (HFS) of the S1 region in Grin1 -vΔ MCx mice did not evoke any significant (F (6,54,63) =0.308; P =0.580) increase in fEPSP slopes in the motor cortex ( Fig. 2d ). In contrast, we observed in Cont -v MCx mice a long-lasting LTP, significantly (F (6,54,63) =11.915; P <0.001) larger than values collected from Grin1 -vΔ MCx mice. In this case, results indicate that the NMDAR is necessary to evoke long-lasting postsynaptic changes in the M1 cortex following HFS of S1 neurons. Synaptic plasticity and the conditioned response Next, we implanted electrodes in Cont -v MCx ( n =10) and Grin1-vΔ MCx ( n =11) mice ( Supplementary Fig. S6 ) to record fEPSPs evoked at the S1–M1 synapse during the classical conditioning of eyelid responses, with an auditory signal as the CS and an electrical shock of the trigeminal nerve as the US [16] , [18] ( Fig. 3a ). After multiple trials of CS–US pairings, an association was formed, enabling a CS alone to elicit a CR, measured by electromyography (EMG) ( Fig. 3b ). 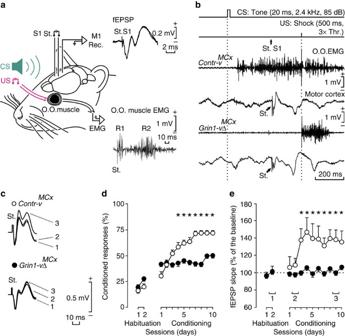Figure 3: Electrophysiological recordings and classical EBC in behaving animals. (a) For classical EBC, animals were implanted with stimulating (St.) electrodes (for US presentation) on the left trigeminal nerve and with electrodes to record (Rec.) the EMG activity of the ipsilateral orbicularis oculi (O.O.) muscle (for recording conditioned responses). The CS consisted of tones delivered from a loudspeaker located 50 cm from the animal’s head. At the top are shown stimulating electrodes implanted in the right primary somatosensory cortex (S1) and recording electrodes implanted in the ipsilateral primary motor cortex (M1). fEPSP evoked in the motor cortex by single pulses applied to the S1 region are illustrated. Corneal reflex responses evoked at the O.O. muscle by electrical stimulation of the trigeminal nerve in aGrin1-vΔMCxmouse are also illustrated. Note the presence of the two (R1, R2) components of the corneal reflex. (b)Grin1-vΔMCxmice were unable of acquiring a conditioned eyeblink response and the accompanying activity-dependent changes in synaptic strength in cortical (S1–M1) synapses asContr-vMCxmice did. From top to bottom are illustrated the conditioning paradigm, representative O.O. EMG and electrocortical recordings during paired CS–US presentations forContr-vMCxandGrin1-vΔMCxmice. The time of S1 stimulation (St. S1) is indicated, as are the times of presentation of CS and US (dotted lines). Data shown were collected during the 9th conditioning session. (c) fEPSPs collected fromContr-vMCx(white circles) andGrin1-vΔMCx(black circles) mice during the conditioning sessions (1–3) indicated in (e). (d) Percentage (mean±s.e.m.) of conditioned responses reached by the two experimental groups (n≥10 per group). Values presented byContr-vMCxmice (white circles) were significantly (*P<0.05, F(1,20,19)=7.800, two-way ANOVA) larger than those reached byGrin1-vΔMCxmice (black circles) from the 4th to the 10th sessions. (e) Evolution of fEPSPs evoked at the S1-primary motor cortex synapse across conditioning for wild-type (white circles) andGrin1-vΔMCx(black circles) mice. Differences in fEPSP slopes (mean±s.e.m.) betweenContr-vMCxand, Grin1-vΔMCxgroups were statistically significant from the 3rd to the 10th conditioning sessions (*P<0.05, F(1,19,18)=8.889, two-way ANOVA). Figure 3: Electrophysiological recordings and classical EBC in behaving animals. ( a ) For classical EBC, animals were implanted with stimulating (St.) electrodes (for US presentation) on the left trigeminal nerve and with electrodes to record (Rec.) the EMG activity of the ipsilateral orbicularis oculi (O.O.) muscle (for recording conditioned responses). The CS consisted of tones delivered from a loudspeaker located 50 cm from the animal’s head. At the top are shown stimulating electrodes implanted in the right primary somatosensory cortex (S1) and recording electrodes implanted in the ipsilateral primary motor cortex (M1). fEPSP evoked in the motor cortex by single pulses applied to the S1 region are illustrated. Corneal reflex responses evoked at the O.O. muscle by electrical stimulation of the trigeminal nerve in a Grin1 -vΔ MCx mouse are also illustrated. Note the presence of the two (R1, R2) components of the corneal reflex. ( b ) Grin1 -vΔ MCx mice were unable of acquiring a conditioned eyeblink response and the accompanying activity-dependent changes in synaptic strength in cortical (S1–M1) synapses as Contr -v MCx mice did. From top to bottom are illustrated the conditioning paradigm, representative O.O. EMG and electrocortical recordings during paired CS–US presentations for Contr -v MCx and Grin1 -vΔ MCx mice. The time of S1 stimulation (St. S1) is indicated, as are the times of presentation of CS and US (dotted lines). Data shown were collected during the 9th conditioning session. ( c ) fEPSPs collected from Contr -v MCx (white circles) and Grin1 -vΔ MCx (black circles) mice during the conditioning sessions (1–3) indicated in ( e ). ( d ) Percentage (mean±s.e.m.) of conditioned responses reached by the two experimental groups ( n ≥10 per group). Values presented by Contr -v MCx mice (white circles) were significantly (* P <0.05, F (1,20,19) =7.800, two-way ANOVA) larger than those reached by Grin1 -vΔ MCx mice (black circles) from the 4th to the 10th sessions. ( e ) Evolution of fEPSPs evoked at the S1-primary motor cortex synapse across conditioning for wild-type (white circles) and Grin1 -vΔ MCx (black circles) mice. Differences in fEPSP slopes (mean±s.e.m.) between Contr -v MCx and, Grin1-vΔ MCx groups were statistically significant from the 3rd to the 10th conditioning sessions (* P <0.05, F (1,19,18) =8.889, two-way ANOVA). Full size image First, we confirmed that reflexively evoked eye blinks collected from Grin1 -vΔ MCx mice were similar from a kinematic point of view to those already described in Cont -v MCx mice [16] ( Fig. 3b ). Control mice ( Cont -v MCx ) acquired the classical conditioning test with a progressive increase in the percentage of CRs, reaching asymptotic values by the 7th conditioning session ( Fig. 3d ). In contrast, Grin1 -vΔ MCx mice presented a non-significant (F (11,99,108) =1.670; P =0.0905) slow increase in the percentage of CRs, reaching values significantly ( P ≤0.05) lower than those presented by the control group from the 4th to the 10th conditioning sessions ( Fig. 3d ). These results indicate that Grin1 -vΔ MCx mice were unable to acquire this type of associative learning task. Interestingly, and in opposition to results collected from Cont -v MCx mice, Grin1-vΔ MCx mice did not present any sign (F (1,19,18) =2.410; P =0.149) of learning-dependent changes in synaptic strength at the S1–M1 synapse ( Fig. 3c and e ). As already reported for hippocampal synapses during classical EBC [16] , the S1–M1 synapse presented a significant ( P <0.05) increase in fEPSP slopes across conditioning. However, in Grin1 -vΔ MCx mice, the increase in fEPSP slopes across conditioning sessions was impaired ( Fig. 3e ). These results indicate that the proper functioning of NMDARs located in the facial motor cortex is necessary both for the acquisition of classical EBC and to evoke the concomitant learning-dependent synaptic plasticity at cortical circuits. Instrumental learning We also checked whether Grin1 -vΔ MCx mice ( n =12) could acquire an instrumental learning task in the same way as their littermate controls ( Cont -v MCx ; n =12). In a first experimental step, animals were trained to acquire a fixed (1:1) ratio schedule—namely, when placed in a Skinner box, they have to learn to obtain a food pellet every time they pressed a lever located nearby the feeder ( Fig. 4a ). Control mice ( Cont -v MCx ) reached the selected criterion (to obtain 20 pellets in 20 min for two successive sessions) slightly (but not significantly; Student’s t -test=−1.746; P =0.096) before the Grin1 -vΔ MCx mice ( Fig. 4b,c ). In a second step, animals were trained to press the lever only when an overlying light bulb was switched on ( Fig. 4a ). Pressing the lever during the dark period was not rewarded and, in addition, delayed the appearance of the lighted period (see Methods). This new conditioning paradigm presented more difficulties to the experimental animals than the early fixed (1:1) ratio schedule. Indeed, Cont -v MCx mice performed this task significantly (F (1,23,11) =17.159; P <0.05) better than Grin1-vΔ MCx mice ( Fig. 4d ), again indicating that NMDAR function in motor cortex circuits is necessary for the acquisition of this type of associative learning task. 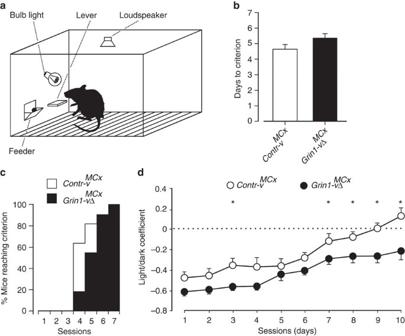Figure 4: Performance during operant conditioning tasks. (a) Experimental set-up. Mice were trained in a Skinner box to press a lever to obtain a food pellet with a fixed-ratio (1:1) schedule. (b) Number of days necessary to reach criterion (mean±s.e.m.) forContr-vMCx(white bar) andGrin1-vΔMCx(black bar) mice. (c) Percentage of mice reaching criterion across training. Note in (b) and (c) thoseContr-vMCxmice (n=10) reached criterion beforeGrin1-vΔMCx(n=11) mice. (d) Performance of the light/dark test. After reaching criterion for a fixed (1:1) schedule, animals were presented with a more difficult task in which lever presses were rewarded only when a light bulb was switched on. In this situation,Contr-vMCxmice presented a significantly (*P≤0.05, two-way ANOVA) better performance thanGrin1-vΔMCxmice. The light/dark coefficient was calculated as: (number of lever presses during the light period−number of lever presses during the dark period)/total number of lever presses (mean±s.e.m.). Figure 4: Performance during operant conditioning tasks. ( a ) Experimental set-up. Mice were trained in a Skinner box to press a lever to obtain a food pellet with a fixed-ratio (1:1) schedule. ( b ) Number of days necessary to reach criterion (mean±s.e.m.) for Contr -v MCx (white bar) and Grin1 -vΔ MCx (black bar) mice. ( c ) Percentage of mice reaching criterion across training. Note in ( b ) and ( c ) those Contr -v MCx mice ( n =10) reached criterion before Grin1 -vΔ MCx ( n =11) mice. ( d ) Performance of the light/dark test. After reaching criterion for a fixed (1:1) schedule, animals were presented with a more difficult task in which lever presses were rewarded only when a light bulb was switched on. In this situation, Contr -v MCx mice presented a significantly (* P ≤0.05, two-way ANOVA) better performance than Grin1 -vΔ MCx mice. The light/dark coefficient was calculated as: (number of lever presses during the light period−number of lever presses during the dark period)/total number of lever presses (mean±s.e.m.). Full size image In the current study, we have developed a combinatorial genetic approach utilizing rAAVs equipped with tet-controlled genetic switches and loxP -engineered knock-in mice for Dox-induced, cell-type-specific Grin1 gene knockout, selectively in the M1 cortex of mice. We provide here very strong evidence that functional loss of the NMDA receptor abolished in vivo LTP in the cortex. We also found that synaptic strengthening of synapses between somatosensory and motor cortices was impaired during associative learning. Importantly, in the same mice, there was strong impairment of conditioned-evoked behavioural responses and learning was significantly reduced in the Skinner-box test. Interestingly, we observed that the Grin1 -vΔ MCx mice showed some residual learning, both in the classical EBC task and the instrumental conditioning. We anticipate two possible explanations for this interesting observation. First, with ~80% of neurons targeted by rAAVs [40] , [41] , and with redundancy in neuronal coding for the same behavioural task in the motor cortex [7] , [42] , possibly to improve behavioural performance [43] , it is possible that the remaining untargeted neurons in the M1 cortex (without the Grin1 gene deletion) might have contributed in executing some residual learning function. Second, it is also possible that in Grin1 -vΔ MCx mice, the cerebellar function, in part, might have participated in trace EBC [44] . Although a simple EBC is a prototypical example of a non-declarative memory, trace and delay EBC are fundamentally different kinds of learning [45] . An introduction of a ‘trace’ [46] component in the EBC endows it with some common features shared with the declarative memory. With dynamic feedforward and top–down interactions between different cortical and subcortical brain regions, involving both localized [15] and widely distributed [47] neuronal networks, distinct cortical cell ensembles representing different experiences might be linked by learning to form unique memories. Our results provide convincing evidence that the memory of acquired trace eyeblink-conditioned responses is localized in the M1 cortex. Therefore, dissecting the mechanisms of trace EBC in the M1 cortex is bound to provide deeper insight into the molecular and cellular mechanisms of declarative memory [48] . Curiously, in earlier studies, genetically modified mice with deletion of the Grin1 gene in CA1 showed deficit in acquisition of both spatial [49] and temporal [50] memories. However, it was later found that, over time (several months), the Grin1 gene deletion in these mice had also spread to all cortical layers [51] , leaving open the possibility that a cortical component might be having a crucial role in forming associations between spatial cues [49] and between temporally separated events [50] . With an improved genetic mouse model, a recent study provides the best evidence thus far that the NMDAR in the dorsal CA1 subfield and dentate gyrus is not required for the acquisition of spatial memories, despite impaired hippocampal LTP in these mice [52] . Instead, hippocampal NMDARs are needed to resolve conflict between competing spatial cues [52] . Notably, deletion of the Grin1 gene specifically in CA3 also did not interfere with trace EBC [53] . However, CA3-NMDARs tend to have a crucial role in the memory of adaptive CR timing [53] . It thus seems quite plausible that while the hippocampus is needed for organizing spatial computations, it is in the cerebral cortex, where spatial memories [49] and temporal associations [50] are acquired and, perhaps, even stored [47] , [54] , [55] , possibly involving both localized and widely distributed cortical cell assemblies [54] . Interestingly, it was found that during classical EBC, the CA3–CA1 synapses and the S1–M1 synapses were similarly strengthened [16] , [18] . As hippocampus lesion is known to impair eyeblink trace conditioning [53] , [56] , it is quite important to investigate the role of CA1-NMDAR function in this particular associative learning paradigm. Our virus-based, chemically controlled genetic approach allows for inducible control of gene expression [34] , [57] and inducible gene knockout in mouse brain. With these powerful tools, it is now possible to precisely manipulate the function of individual neuronal cell types, cortical layers and brain regions in different mammalian species. In our current study, the AAVs of hybrid serotype 1 and 2 targeted cortical neurons [40] , [41] of layer 2/3 and layer 5, thereby deleting in these cells the Grin1 gene and impairing NMDAR function. In future studies, our virus-based inducible genetic approach should further help to investigate, in cortical layer- and cell-type-specific manner, whether motor cortex NMDAR function is required for consolidation and retrieval of the conditioned eyeblink response. Motor cortex-specific Grin1 gene knockout Homozygous Grin1 2loxP mice or ( Grin1 tm1Rsp ) [33] were generated by mating heterozygous males with heterozygous females. Viruses equipped with tet-controlled genetic switches [34] , [57] were bilaterally injected in the primary motor cortex (M1) of adult homozygous Grin1 2loxP male [33] mice or wild-type control ( Contr ) littermates, and abbreviated as Grin1 -v MCx and Contr -v MCx , respectively. Three weeks after virus (v) injection, both groups of mice were similarly treated with Dox, enabling Cre-mediated deletion (Δ) of the Grin1 gene in adult homozygous Grin1 2loxP males [33] and leading to the generation of motor cortex (MCx)-specific Grin1 gene knockout mice (here referred to as Grin1 -vΔ MCx ). These mice were analysed for Dox-induced gene expression, Grin1 gene deletion by in situ hybridization and functional NMDAR activity. See Supplementary Methods for details on the combinatorial genetic approach applied for motor cortex-specific Grin1 gene knockout in the mouse brain and for validating functional loss of Grin1 gene expression by in situ hybridization, and NMDA receptor function by in vitro electrophysiology. All experiments were conducted according to German and Spanish animal welfare regulations. Surgery for chronic-recording experiments Animals were anesthetized with 0.8–3% halothane delivered from a calibrated Fluotec 5 (Fluotec-Ohmeda, Tewksbury, Massachusetts, USA) vaporizer at a flow rate of 1–2 l min −1 oxygen. Animals were implanted with bipolar stimulating electrodes aimed at the facial area [18] of the right S1 region (1 mm posterior to bregma, 2.5 mm lateral and 1.2 mm from brain surface) and with two recording electrodes aimed at the facial [18] ipsilateral primary motor cortex (1 mm anterior to bregma, 1 mm lateral and 0.8 mm from brain surface). These electrodes were made of 50 μm, Teflon-coated tungsten wire (Advent Research Materials Ltd, Eynsham, UK). The final position of the recording electrodes was determined using as a guide the field potential depth profile evoked by paired (40 ms of interval) pulses presented at the S1 area [18] . A bare silver wire (0.1 mm) was affixed to the skull as a ground. Wires were connected to a four-pin socket and the socket was fixed to the skull with the help of two small screws and dental cement [16] . Recording and stimulation procedures Both the EMG activity of the orbicularis oculi muscle and fEPSPs were recorded with Grass P511 differential amplifiers (Grass-Telefactor, West Warwick, Rhode Island, USA), at a bandwidth of 0.1 Hz–10 kHz. A high-impedance probe (2 × 10 12 Ω, 10 pF) was used for fEPSP recordings. Electrical stimulus applied to the S1 region consisted of 100 μs, square, biphasic pulses presented alone, paired or in trains. Stimulus intensities ranged from 0.02 to 0.4 mA for the construction of the input/output curves. For paired-pulse facilitation, the stimulus intensity was set well below the threshold for evoking a population spike, usually 30–40% of the intensity (mA) necessary for evoking a maximum fEPSP response [58] . Paired pulses were presented at six (10, 20, 40, 100, 200 and 500 ms) different pulse intervals. For LTP induction, the stimulus intensity was also set at ≈35% of peak fEPSP values. An additional criterion for selecting stimulus intensity for LTP induction was that a second stimulus, presented 40 ms after a conditioning pulse, evoked a synaptic field potential 20% larger than the first fEPSP [59] . After 15 min of baseline records (1 stimulus per 20 s), each animal was presented with an HFS protocol consisting of five trains (200 Hz, 100 ms) of pulses at a rate of 1 per s. This protocol was presented six times in total, at intervals of 1 min. Evolution of fEPSPs after the HFS protocol was followed for 30 min at the same stimulation rate (1 stimulus per 20 s). Additional recording sessions (15 min) were carried out for up to 5 days [16] , [38] . Classical EBC Experimental sessions were carried out with three animals at a time. Animals were placed in separate small (5 × 5 × 10 cm) plastic chambers located inside a larger (30 × 30 × 20 cm) Faraday box. Animals were classically conditioned using a trace paradigm. For this, a tone (20 ms, 2.4 kHz, 85 dB) was presented as CS, while the US consisted of a 500-μs, 3 × threshold, square, cathodal pulse applied to the supraorbital nerve 500 ms after the end of the CS. A total of two habituation and 10 conditioning sessions (one session per day) were carried out for each animal. A conditioning session consisted of 60 CS–US presentations, and lasted for ≈30 min. For a proper analysis of conditioned responses, the CS was presented alone in 10% of the cases. CS–US presentations were separated at random by 30±5 s. For habituation sessions, only the CS was presented, also for 60 times per session, at intervals of 30±5 s. As a criterion, we considered a ‘conditioned response’, the presence, during the CS–US interval, of EMG activity lasting >20 ms and initiated >50 ms after CS onset. In addition, the integrated EMG activity recorded during the CS–US interval had to be at least 2.5 times greater than the averaged activity recorded immediately before CS presentation [16] , [60] . During habituation and conditioning sessions, fEPSPs were evoked in the motor cortex area by single 100 μs, square, biphasic (negative–positive) pulses applied the S1 region 300 ms after CS presentation. As above-indicated, pulse intensity was set at 30–40% of the amount necessary to evoke a maximum fEPSP response (range, 0.05–0.15 mA). An additional criterion for selecting stimulus intensity was that a second stimulus, presented 40 ms later, evoked a larger (>20%) synaptic field potential than the first [38] , [59] . Instrumental conditioning Training and testing took place in five Skinner box modules measuring 12.5 × 13.5 × 18.5 cm (MED Associates, St Albans, Vermont, USA). The operant conditioning boxes were housed within independent sound-attenuating chambers (90 × 55 × 60 cm), which were constantly illuminated (19 W lamp) and exposed to a 45 dB white noise (Cibertec SA, Madrid, Spain). Each Skinner box was equipped with a food dispenser from which pellets (Noyes formula P; 45 mg; Sandown Scientific, Hampton, UK) could be delivered by pressing a lever. Before training, mice were handled daily for 7 days and food-deprived to 80% of their free-feeding weight. Training took place for 20 min during successive days, in which mice were allowed to press the lever to receive pellets from the feeder using a fixed-ratio (1:1) schedule. The start and end of each session was indicated by a tone (2 kHz, 200 ms, 70 dB) provided by a loudspeaker located in the isolating chamber. Animals were maintained on this 1:1 schedule until they reached the selected criterion—namely, until they were able to obtain ≥20 pellets for two successive sessions. Mice reached the criterion after 4–7 days of training. Once the criterion for the 1:1 schedule was reached, conditioning was carried out for 10 additional days using a light/dark protocol. In this protocol, only lever presses performed during the light period (20 s) were reinforced with a pellet. In contrast, lever presses performed during the dark period (20±10 s) were not reinforced. Moreover, lever presses carried out during the dark period increased its duration in up to 10 additional seconds. Histology At the end of the recording sessions, mice were deeply anesthetized (sodium pentobarbital, 50 mg kg −1 ) and perfused transcardially with saline and 4% phosphate-buffered paraformaldehyde. Brains were dissected, postfixed overnight at 4 °C, and cryoprotected in 30% sucrose in PBS. Sections were obtained in a microtome (Leica, Wetzlar, Germany) at 50 μm. Some selected sections including motor and somatosensory cortices were mounted on gelatinized glass slides and stained using the Nissl technique with 0.1% toluidine blue to determine the location of stimulating and recording electrodes. Data analysis Field EPSPs, EMG and 1-V rectangular pulses corresponding to CS and US presentations were stored digitally on a computer via an analogue/digital converter (CED 1401 Plus, Cambridge, England) at a sampling frequency of 11–22 kHz and with an amplitude resolution of 12 bits. Data were analysed offline for quantification of conditioned responses and fEPSP slopes with the help of commercial (Spike 2 and SIGAVG from CED) and custom programs [16] , [60] . The slope of evoked fEPSPs was computed as the first derivative (V s −1 ) of fEPSP recordings (V). For this, five successive fEPSPs were averaged, and the mean value of the slope during the rise time period (that is, between the initial and final 10% of the fEPSP) was determined. Computed results were processed for statistical analysis using the Sigma Stat software package (SSI, San Jose, California). Instrumental conditioning programs, lever presses and delivered reinforcements were controlled and recorded by a computer, using a MED-PC programme (MED Associates). Operant sessions were recorded with a synchronized video capture system (Sony HDR-SR12E, Tokyo, Japan) for offline analysis. How to cite this article: Hasan Mazahir T. et al . Role of motor cortex NMDA receptors in learning-dependent synaptic plasticity of behaving mice. Nat. Commun. 4:2258 doi: 10.1038/ncomms3258 (2013).